Cadherin selectivity filter regulates endothelial sieving properties The molecular basis of endothelial protein sieving, the critical vascular barrier function that restricts flow of large plasma proteins into tissues while allowing small molecules and water to pass, is not understood. Here, we address this issue using a novel assay to detect macromolecular penetrance at microdomains of endothelial adherens junctions. Adherens junctions, as detected by cadherin-GFP expression, were distributed in the cell perimeter as high- or low-density segments. Low but not high-density segments permitted penetrance of a 70-kDa fluorescent dextran, a molecule of equivalent size to albumin. Expression of a cadherin mutant that abrogates strand–swap adhesive binding in the cadherin EC1 ectodomain, or alternatively of an α-actinin-1 mutant that inhibits F-actin bundling, increased both cadherin mobility and 70 kDa dextran penetrance at high-density segments. These findings suggest that adhesive interactions in the cadherin EC1 domain, which underlie adherens junction structure, are critical determinants of endothelial macromolecular sieving. Microvascular fluid filtration is a process in which regulated transvascular leak of water and proteins takes place to maintain tissue hydration, lymph flow and immune defence. During filtration, the endothelial barrier sieves proteins, allowing transport of small but not large proteins such as albumin [1] , [2] . The resulting protein gradient—with higher concentrations in plasma than tissue—establishes the plasma oncotic pressure, which is critical for retention of vascular water and maintenance of blood volume [3] , [4] . Failure of endothelial sieving in diseases, such as sepsis, metastatic cancer and developmental anomalies can cause vascular hyperpermeability and hyperfiltration, leading to life-threatening oedemas [5] , [6] . Because of the physiological importance of these processes, the molecular basis of endothelial protein sieving requires better understanding. Adherens junctions (AJs) have been implicated in the maintenance of the endothelial barrier [7] , [8] . AJs are formed by the transmembrane cadherins; VE-cadherin in human and mouse [9] , [10] , [11] and E-cadherin in rat [12] , [13] , [14] . Cadherins are stabilized by trans interactions that establish cell–cell adhesion and by cis interactions that are important for packing the protein in AJs [15] , [16] , [17] , [18] . Cadherins contain five tandem extracellular cadherin domains (ECs) in their ectodomains, EC1–EC5, and a cytoplasmic domain that binds β-catenin [19] that in turn binds α-catenin [16] , [20] which links the cadherin complex to actin. Exposure of endothelial monolayers to antibodies against EC domains [21] , [22] , or expression of mutant cadherins lacking the ectodomain or the β-catenin-binding site, induces endothelial hyperpermeability [23] . However, endothelial barrier effects of mutations specific to the EC1 domain, the site of cell-adhesive trans interactions [24] , [25] , [26] , remain unknown. The cell-to-cell adhesive interactions of classical cadherins are mediated by 'strand–swap' interactions in which the N-terminal β-strands of partner EC1 domains from apposed cells exchange bound positions to form a dimer interface [24] , [26] , [27] . The swap interaction is anchored by the insertion of the side chain of the conserved tryptophan (W2) residue of one EC1 domain in a hydrophobic pocket in the partner EC1 domain [24] , [27] . Expression of the W2-to-alanine (W2A) mutation inhibits strand swapping, which inhibits adhesion for all classical cadherins. CHO cells expressing the W2A mutant fail to aggregate in the shaking-bath assay [24] , [26] , suggesting that strand–swap dimerization in the EC1 ectodomain is critical for cell adhesion. For cadherin lacking cytosolic linkages, the W2A mutation increases cadherin mobility in epithelial cells [28] , pointing to the importance of trans interactions in corralling cadherin at AJs. Hence, EC1 strand–swap interactions might have a role in determining sieving properties of the endothelial barrier. A cadherin endothelial barrier would also be likely to be dependent on cadherin tethering in the cytosol. It has been proposed that the binding of α-catenin to F-actin forms such a tether [29] , [30] . This view is supported by evidence that cadherin mobility increases in epithelial AJs following knockdown of α-catenin [31] . According to the opposite view, the mobility was unaffected by expression of a mutant cadherin lacking the cytoplasmic domain, or of a mutant α-catenin lacking the linkage with F-actin [32] . Endothelial cells express α-actinin-1 and –4, which are implicated in the barrier-enhancing effect of the lipid growth factor, sphingosine-1 phosphate [33] . α-actinin-1 is constitutively expressed at AJs [34] , [35] as different from α-actinin-4, which localizes on stress fibres in the cytosol and subserves cell motility [36] . α-actinin-1 contains an F-actin-binding site at the N-terminal domain [37] and an α-catenin-binding site in the spectrin repeat domain [34] , [35] , [37] , suggesting that these sites might provide cadherin's tether linkages to F-actin. We tested the effects of interfering with AJ structure, both by the direct W2A E-cadherin mutation and by interfering with cytoskeletal linkage, on macromolecular penetrance and cadherin mobility in endothelial AJs. Our results are consistent with the idea that macromolecular penetrance depends on properties of AJs as determined by cadherin adhesive binding and by tethering to F-actin. AJs distribute as high- and low-density clusters In wild-type (WT) endothelial monolayers, AJ distribution, as reflected by immunofluorescence of endogenous cadherin, was markedly uneven, varying almost twofold between different locations ( Fig. 1a,b ). This distribution was different from that of 'spot AJs' in epithelia [31] , [38] in that here, patches of high-density AJs (HAJs) were distributed as non-contiguous segments ( Fig. 1b ). Together, HAJs comprised 65±5% of the junctional perimeter. In remaining perimeter regions, which we termed low-density AJs (LAJs), cadherin density was spotty ( Fig. 1a,b ). Z axis imaging revealed that E-cadherin was highly clustered throughout the paracellular pathway of HAJs. As junctional width is in the nanometre scale, the micrometre thickness of the cadherin band suggests the presence of junctional folds that integrated the fluorescence. By contrast, at LAJs the Z axis cadherin distribution was weak ( Supplementary Fig. S1 ). 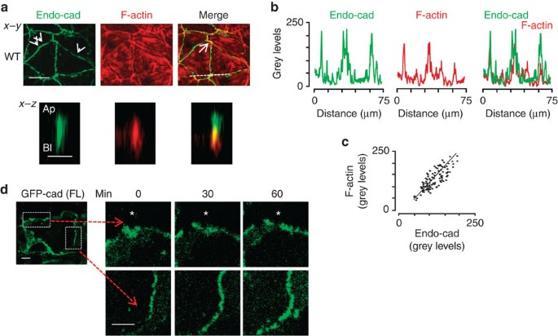Figure 1: Cadherin distribution in endothelial junctions. (a–c) Confocal images of WT endothelial monolayers show immunofluorescence (IF) of indicated proteins. (a). High-density (double arrowhead) and low-density (single arrowhead) AJs are indicated. The merged panel shows the locus (arrow) at which images were obtained for thex–zprojections . Endo-cad, endogenous E-cadherin; Ap, apical; BI, basolateral. Scale bars are 40 μm (x–yimages) and 8 μm (x–zimages). Fluorescence intensities determined along the junction-intersecting line shown in the merged image (dashes) are indicated by the tracings (b) and as a group plot (c). Line in group plot is drawn by linear regression (P<0.01; data are for 60–80 cells from five monolayers). (d) Confocal images show time-dependent changes of GFP fluorescence in a non-confluent monolayer expressing GFP-E-cadherin (GFP-cad). The monolayer was grown for 48 h before imaging. The enlarged time-lapse images show regions demarcated by the dotted lines in which cadherin fluorescence spontaneously decreased (star in upper panels) or increased (lower panels). Scale bars, 5 μm. Replicated in five monolayers. Figure 1: Cadherin distribution in endothelial junctions. ( a – c ) Confocal images of WT endothelial monolayers show immunofluorescence (IF) of indicated proteins. ( a ). High-density (double arrowhead) and low-density (single arrowhead) AJs are indicated. The merged panel shows the locus (arrow) at which images were obtained for the x – z projections . Endo-cad, endogenous E-cadherin; Ap, apical; BI, basolateral. Scale bars are 40 μm ( x – y images) and 8 μm ( x – z images). Fluorescence intensities determined along the junction-intersecting line shown in the merged image (dashes) are indicated by the tracings ( b ) and as a group plot ( c ). Line in group plot is drawn by linear regression ( P <0.01; data are for 60–80 cells from five monolayers). ( d ) Confocal images show time-dependent changes of GFP fluorescence in a non-confluent monolayer expressing GFP-E-cadherin (GFP-cad). The monolayer was grown for 48 h before imaging. The enlarged time-lapse images show regions demarcated by the dotted lines in which cadherin fluorescence spontaneously decreased (star in upper panels) or increased (lower panels). Scale bars, 5 μm. Replicated in five monolayers. Full size image As F-actin is implicated in AJ stability [31] , [39] , [40] , we visualized the cortical cytoskeletal organization in endothelial monolayers. In WT cells, F-actin density varied directly with AJ density ( Fig. 1a–c ). Projections of HAJ images in the depth ( x – z ) axis indicated that F-actin and cadherin best co-localized on the basolateral aspect ( Fig. 1a ). Further, F-actin, and α- and β-catenins co-distributed in HAJs and LAJs in proportion to cadherin density ( Supplementary Fig. S2a,b ). Thus, our findings indicate that the density distributions of the catenins corresponded to the cadherin density distribution. AJ remodelling in growing monolayers To determine whether LAJs can transform to HAJs, we obtained time-lapse images of monolayers grown at low and high densities of endothelial cells expressing GFP-E-cadherin (GFP-cad). The non-confluent, low-density monolayers were grown for 48 h after cell seeding, whereas confluent monolayers were grown for 72 h. In non-confluent monolayers, spontaneous time-dependent changes of cadherin fluorescence were clearly evident at different regions of the endothelial perimeter. In some regions, the fluorescence progressively increased, whereas at others it decreased ( Fig. 1d ). By contrast, no spontaneous fluorescence changes were evident in confluent monolayers (not shown). These findings indicate that under conditions in which the endothelial junction remodels, as in the non-confluent monolayers, LAJs transform to form HAJs and vice versa. These findings affirm that the unit composition of the cadherin complex is essentially the same at LAJs and HAJs. The W2A mutation maintains F-actin distribution To determine whether interference with the strand–swap interactions changes F-actin distribution, we expressed the W2A mutant of GFP-cad in endothelial cells. For control, we expressed full-length GFP-cad. To confirm that the exogenous GFP-cad was surface expressed, we carried out immunoblots on biotin-exposed samples of the monolayers to recover surface proteins. These immunoblots indicated that the band for GFP-cad was upward shifted from the band for endogenous E-cadherin ( Fig. 2a ). This band shift, which is consistent with the higher molecular weight of GFP-cad, identified the extents to which the exogenous and endogenous E-cadherins were expressed in these transfected cells. Immunoblots for GFP confirmed that the upper band represented exogenous E-cadherin ( Fig. 2a ). According to the immunoblot data, total endogenous cadherin decreased in W2A-overexpressing cells ( Fig. 2a ; Supplementary Fig. S3 ). However, the imaging data indicate that similar levels of endogenous cadherin were localized at HAJs in non-transfected ( Fig. 1a ) and W2A-overexpressing ( Fig. 2b ) cells. There was therefore, no loss of endogenous cadherin from the HAJs of W2A-overexpressing cells. The transfection was stable, as GFP-cad expression could be confirmed in passaged endothelial cells. The distribution of GFP-cad matched that of the endogenous protein, indicating that the cadherin density variation was a constitutive feature of the endothelial cell ( Supplementary Fig. S1 ). By fluorescence microscopy, we confirmed that GFP-cad was present in all cells of monolayers grown with the transfected cells ( Supplementary Fig. S3 ). 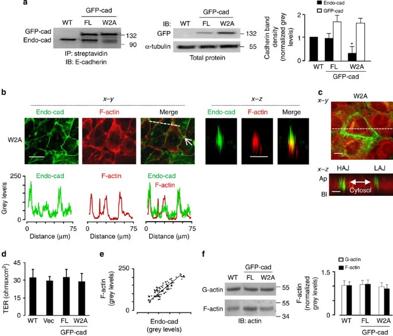Figure 2: Cadherin and F-actin co-distribution in endothelial junctions. Data for WT monolayers, and monolayers transfected with full-length (FL) or mutant (W2A) E-cadherin. (a) The data are for endothelial cell surface proteins. Intact monolayers were exposed to biotin, immunoprecipitated (IP) with streptavidin, then immunoblotted (IB) as indicated. Left panel shows expression of exogenous GFP-E-cadherin (GFP-cad) and endogenous cadherin (Endo-cad). Note, only endogenous cadherin is present in WT cells. Right panel shows GFP expression was present in monolayers expressing full-length or mutant E-cadherin. IB with α-tubulin indicates protein loading was equal in all lanes. The density analyses are normalized to WT. *P<0.01 compared with WT by one-way ANOVA. (b) Confocal images of endothelial monolayers expressing mutant W2A show immunofluorescence (IF) of indicated proteins. The indicated location in the merge panel (arrow) is the site of thex–zprojections. Fluorescence intensities determined along the linear junction-intersecting line in the merged image (dashes) are shown as tracings. Endo-cad, endogenous E-cadherin; Ap, apical; BI, basolateral. Scale bars are 40 μm (x–yimages) and 8 μm (x–zimages). (c) Images of an endothelial monolayer show expression of the GFP-expressing W2A mutant as fluorescence (green) distribution. The dashed line shows the axis at which thex–zimages were obtained. The calcein-loaded cytosol is shown in red (double-headed arrow). Scale bar, 10 μm. (d) The bar diagram shows trans-endothelial electrical resistance (TER) for endothelial monolayers. Vec, vector. Data are mean±s.e.m. from four monolayers in each group. (e) The line was drawn by linear regression analysis.P<0.01, data are for 60–80 cells from five monolayers. (f) Immunoblot (IB) on endothelial cell lysates and quantifications of band density are shown for triton-soluble (G-actin) and -insoluble (F-actin) fractions. *P<0.01 compared with WT by one-way ANOVA. All protein data are normalized to WT. Data are mean±s.e.m.n=5monolayers for each bar. Figure 2: Cadherin and F-actin co-distribution in endothelial junctions. Data for WT monolayers, and monolayers transfected with full-length (FL) or mutant (W2A) E-cadherin. ( a ) The data are for endothelial cell surface proteins. Intact monolayers were exposed to biotin, immunoprecipitated (IP) with streptavidin, then immunoblotted (IB) as indicated. Left panel shows expression of exogenous GFP-E-cadherin (GFP-cad) and endogenous cadherin (Endo-cad). Note, only endogenous cadherin is present in WT cells. Right panel shows GFP expression was present in monolayers expressing full-length or mutant E-cadherin. IB with α-tubulin indicates protein loading was equal in all lanes. The density analyses are normalized to WT. * P <0.01 compared with WT by one-way ANOVA. ( b ) Confocal images of endothelial monolayers expressing mutant W2A show immunofluorescence (IF) of indicated proteins. The indicated location in the merge panel (arrow) is the site of the x – z projections. Fluorescence intensities determined along the linear junction-intersecting line in the merged image (dashes) are shown as tracings. Endo-cad, endogenous E-cadherin; Ap, apical; BI, basolateral. Scale bars are 40 μm ( x – y images) and 8 μm ( x – z images). ( c ) Images of an endothelial monolayer show expression of the GFP-expressing W2A mutant as fluorescence (green) distribution. The dashed line shows the axis at which the x – z images were obtained. The calcein-loaded cytosol is shown in red (double-headed arrow). Scale bar, 10 μm. ( d ) The bar diagram shows trans-endothelial electrical resistance (TER) for endothelial monolayers. Vec, vector. Data are mean±s.e.m. from four monolayers in each group. ( e ) The line was drawn by linear regression analysis. P <0.01, data are for 60–80 cells from five monolayers. ( f ) Immunoblot (IB) on endothelial cell lysates and quantifications of band density are shown for triton-soluble (G-actin) and -insoluble (F-actin) fractions. * P <0.01 compared with WT by one-way ANOVA. All protein data are normalized to WT. Data are mean±s.e.m. n=5 monolayers for each bar. Full size image In monolayers expressing the W2A mutant, the distributions of HAJs and LAJs ( Fig. 2c ) as well as of GFP-cad expression, as indicated by immunoblots ( Fig. 2a ), were similar to that in monolayers expressing the full-length GFP-cad. The immunoblots indicated that endogenous cadherin in the transfected cells was lower than WT. The mutant did not alter the transendothelial electrical resistance, a measure of the overall integrity of the monolayer ( Fig. 2d ), indicating that the reduction of endogenous cadherin did not deteriorate the monolayer. The HAJ association with F-actin was unchanged from that of WT cells ( Fig. 2b,e ). Immunoblots indicated that the W2A mutant did not alter the F/G actin ratio ( Fig. 2f ). To determine this ratio, we used the two-stage solubilizing approach [12] , to sequentially extract G- and then F-actin. These studies indicated that the W2A mutation did not diminish cortical F-actin density. Hence, inhibition of the strand–swap interactions did not affect the distribution of the cortical actin cytoskeleton. The Y12F mutation abrogates F-actin distribution at HAJs As α-actinin-1 binds actin in the N-terminal domain-containing tyrosine at position 12 (Y12), we expressed a mutant α-actinin-1 (Y12F) in which Y12 was replaced by phenyalanine. As expected, this mutation decreased tyrosine phosphorylation of α–actinin–1 ( Fig. 3a ). The Y12F mutation did not affect membrane cadherin expression ( Fig. 3b ), but it markedly decreased actin density in the monolayer as indicated by decreased F-actin fluorescence ( Fig. 3c ), by loss of co-association of F-actin with the HAJs ( Fig. 3d ) and by decreased F-actin expression in immunoblots ( Fig. 3e ). In WT monolayers, density distributions for cortical F-actin and α-actinin-1 matched the cadherin distribution ( Fig. 3f ), indicating that actin bundling was greatest at HAJs. The Y12F mutation decreased the co-distribution of α-actinin-1 with F-actin ( Fig. 3g ). 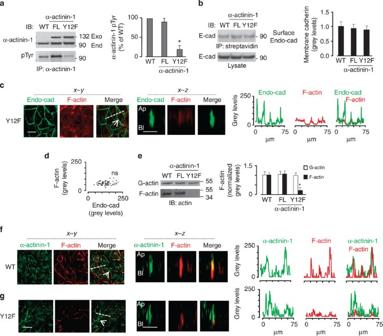Figure 3: Association of α-actinin-1 and F-actin in endothelial junctions. Data for WT monolayers, and monolayers transfected with full-length (FL) or mutant (Y12F) α-actinin-1 were obtained by immunoprecipitation (IP) followed by immunoblot (IB) (a,b) or by confocal imaging of immunofluorescence (IF) (c–g). Bars show density analyses. (a) The IBs indicate that the transfected monolayers expressed both exogenous and endogenous α-actinin-1. Note, tyrosine phosphorylation (pTyr) was reduced in Y12F-expressing monolayers. *P<0.005 compared with WT by one-way ANOVA. (b) The data are for endothelial cell surface proteins. Intact monolayers were exposed to biotin, IP with streptavidin, then IB as indicated. (c–g) Thex–zprojections were obtained at the indicated sites (arrows). Fluorescence intensities determined along the junction-intersecting lines shown in the merged images (dashes) are indicated as tracings. Thex-axes of the tracings are distances along the junction-intersecting lines. Ap, apical; BI, basolateral. The IF (c) indicates co-distribution of endogenous cadherin (endo-cad) and F-actin for the Y12F mutant inx–y(left panels) andx–zprojections (right panels). The fluorescence intensities are plotted (d). IB on endothelial lysates and quantifications of band densities are shown for triton-soluble (G-actin) and -insoluble (F-actin) fractions (e). *P<0.01 compared with WT by one-way ANOVA. IF indicates co-distribution of endogenous α-actinin-1 and F-actin for WT (f) and for the mutant (Y12F) (g) in thex–yandx–zplanes. Scale bars are 40 μm inx–yimages and 8 μm inx–zimages. All densitometric analyses are normalized to WT. Data are mean±s.e.m.n=5 monolayers for each bar. Figure 3: Association of α-actinin-1 and F-actin in endothelial junctions. Data for WT monolayers, and monolayers transfected with full-length (FL) or mutant (Y12F) α-actinin-1 were obtained by immunoprecipitation (IP) followed by immunoblot (IB) ( a , b ) or by confocal imaging of immunofluorescence (IF) ( c – g ). Bars show density analyses. ( a ) The IBs indicate that the transfected monolayers expressed both exogenous and endogenous α-actinin-1. Note, tyrosine phosphorylation (pTyr) was reduced in Y12F-expressing monolayers. * P <0.005 compared with WT by one-way ANOVA. ( b ) The data are for endothelial cell surface proteins. Intact monolayers were exposed to biotin, IP with streptavidin, then IB as indicated. ( c – g ) The x – z projections were obtained at the indicated sites (arrows). Fluorescence intensities determined along the junction-intersecting lines shown in the merged images (dashes) are indicated as tracings. The x -axes of the tracings are distances along the junction-intersecting lines. Ap, apical; BI, basolateral. The IF ( c ) indicates co-distribution of endogenous cadherin (endo-cad) and F-actin for the Y12F mutant in x – y (left panels) and x – z projections (right panels). The fluorescence intensities are plotted ( d ). IB on endothelial lysates and quantifications of band densities are shown for triton-soluble (G-actin) and -insoluble (F-actin) fractions ( e ). * P <0.01 compared with WT by one-way ANOVA. IF indicates co-distribution of endogenous α-actinin-1 and F-actin for WT ( f ) and for the mutant (Y12F) ( g ) in the x – y and x – z planes. Scale bars are 40 μm in x – y images and 8 μm in x – z images. All densitometric analyses are normalized to WT. Data are mean±s.e.m. n= 5 monolayers for each bar. Full size image Cadherin mobility at AJs To determine the effect of different actin densities on HAJ stability, we carried out cadherin mobility assays in monolayers expressing cadherin-GFP. Consistent with studies in epithelia [31] , in WT monolayers, cadherin mobility occurred with an apparent diffusion coefficient of 3–6×10 −3 μm 2 s −1 . The mobility related inversely to cadherin density, being higher at LAJs than at HAJs ( Fig. 4a–i ). Kymograph analyses confirmed that fluorescence recovery was attributable to cadherin diffusion within the membrane, rather than diffusion from the cytosol to the membrane ( Fig. 4j ). Among different junctional microdomains, the cadherin mobile fraction was least at HAJs ( Fig. 4k ), suggesting that cadherin tethering was best developed at sites of increased F-actin density. Increases of the cadherin mobile fraction in W2A-expressing monolayers, in which F-actin was unchanged, were similar to those in Y12F-expressing monolayers in which F-actin was reduced ( Fig. 4k ). We interpret from these results that cadherin mobility, a measure of cadherin tethering, was determined by strand–swap interactions in the EC1 ectodomain as well as by actin density. 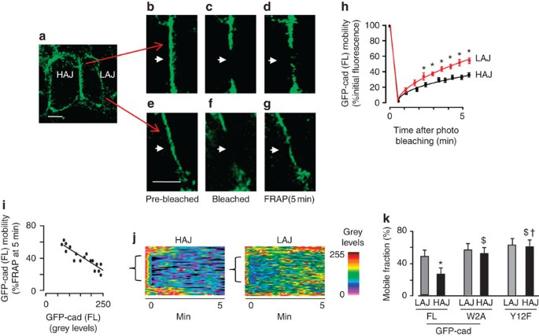Figure 4: FRAP determinations of cadherin mobility in endothelial junctions. (a–g) Endothelial cells of a monolayer (a) show full-length GFP-cad expression in low-density (LAJ) and high-density (HAJ) adherens junctions. High magnification views (b–g) of the indicated regions (red arrows) are shown before (b,e) and immediately after (c,f) photobleaching. In the subsequent 5 min, FRAP was poor at the HAJ (d), but well developed at the LAJ (g). Scale bars, 10 μm (e). (h,i) Plots (h) show GFP-cad mobility rates at high density (HAJ) and low density (LAJ). FRAP is calculated as percentage of the initial fluorescences. ANOVA with Newman Keulspost-hocanalysis was used for LAJ versus HAJ comparisons for each time point. *P<0.01 compared withHAJ.The line (i) was calculated by the regression of GFP-cad mobility against GFP-cad density along the endothelial perimeter (P<0.05). For all data, each point is mean±s.e.m. for 50 cells from five monolayers. (j) Kymographs show FRAP profiles for the HAJ (left) and the LAJ (right) shown in the images. The indicated regions (brackets) show fluorescence before (red) and after (blue) bleaching, and the subsequent fluorescence recovery in pseudocolours corresponding to different grey levels. (k) The bars show mobile fractions for different groups. Data are mean±s.e.m. for 50 cells from five monolayers for each group. * and †P<0.001 compared with LAJ in the WT group.$P<0.001 compared with HAJ in the WT group. ANOVA with Newman Keulspost-hocanalyses was used for comparisons. Figure 4: FRAP determinations of cadherin mobility in endothelial junctions. ( a – g ) Endothelial cells of a monolayer ( a ) show full-length GFP-cad expression in low-density (LAJ) and high-density (HAJ) adherens junctions. High magnification views ( b – g ) of the indicated regions (red arrows) are shown before ( b , e ) and immediately after ( c , f ) photobleaching. In the subsequent 5 min, FRAP was poor at the HAJ ( d ), but well developed at the LAJ ( g ). Scale bars, 10 μm ( e ). ( h , i ) Plots ( h ) show GFP-cad mobility rates at high density (HAJ) and low density (LAJ). FRAP is calculated as percentage of the initial fluorescences. ANOVA with Newman Keuls post-hoc analysis was used for LAJ versus HAJ comparisons for each time point. * P <0.01 compared with HAJ. The line ( i ) was calculated by the regression of GFP-cad mobility against GFP-cad density along the endothelial perimeter ( P <0.05). For all data, each point is mean±s.e.m. for 50 cells from five monolayers. ( j ) Kymographs show FRAP profiles for the HAJ (left) and the LAJ (right) shown in the images. The indicated regions (brackets) show fluorescence before (red) and after (blue) bleaching, and the subsequent fluorescence recovery in pseudocolours corresponding to different grey levels. ( k ) The bars show mobile fractions for different groups. Data are mean±s.e.m. for 50 cells from five monolayers for each group. * and † P <0.001 compared with LAJ in the WT group. $ P <0.001 compared with HAJ in the WT group. ANOVA with Newman Keuls post-hoc analyses was used for comparisons. Full size image Macromolecular sieving at AJs To test the possibility that AJ structure determined barrier permeability, it was important to quantify macromolecular penetrance at HAJs. As no approaches are available for quantifying domain-specific cell junctional permeability, we developed a new method using apically added fluorescent dextran of different molecular sizes as transport markers and z axis imaging to detect dextran penetrance at specific junctional locations. The junctional cleft was exactly localized by cadherin fluorescence ( Fig. 5a ) and accumulation of dextran fluorescence in the cleft quantified macromolecular penetrance. The dextrans were of molecular size 4 (D4), 20 (D20) and 70 kDa (D70) to approximately model small, medium and large plasma proteins. In the x – z image projection, junctional penetrance of FD4 was rapid at both LAJs than HAJs ( Fig. 5b ). At both locations, D4 fluorescence could be visualized at junctional exits on the basolateral aspect of the cell. By contrast, the junctional penetrance of D20 was faster at LAJs than HAJs ( Fig. 5c ). D70 also penetrated the LAJs, but at a rate slower than for D20, indicating that even at LAJs, there was substantial size-dependent selectivity of macromolecular penetrance. By contrast at HAJs, D70 penetrance was negligible ( Fig. 5b–d ), although D20 penetrance was evident, albeit at levels lower than at LAJs ( Fig. 5d ). These findings indicate that the endothelial barrier sieved macromolecules at both LAJs and HAJs, but that HAJs were much more restrictive to D70 transit. 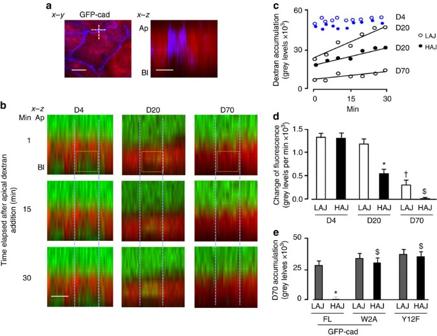Figure 5: Dextran permeation through endothelial adherens junctions. (a,b) Confocal images of WT endothelial monolayers show dextran permeation. (a) The left image shows anx–yprojection of an endothelial cell of a monolayer expressing full-length GFP-cad (blue pseudocolor). The cytosol is stained with calcein red. The right image shows thex–zprojection of an HAJ identified at the cross-hairs on the left image. Ap, apical; BI, basolateral. (b) After layering dextran of 4 (D4), 20 (D20) or 70 (D70) kDa (green) on the apical surface, fluorescence accumulation in thex–zplane was imaged over time. D4 and D20, but not D70 penetrated the HAJ. Red pseudocolor denotes the cytosol. Rectangles show sites of analyses for dextran fluorescence in the junctional cleft. (c,d) Plots from single AJs and the group data show time course of dextran accumulation. Scale bars are 10 μm (x–yimages) and 2 μm (x–zimages). *P<0.005 compared with HAJ of D4, †P<0.005 compared with LAJ of D20 and $P<0.005 compared with HAJ of D20. (e) Group data for LAJs and HAJs show D70 penetrance at 30 min for monolayers transfected with full-length (FL) or mutant (W2A) E-cadherin or with the α-actinin-1 mutant (Y12F). *P<0.002 compared with left bar.$P<0.002 compared with HAJ in WT group. ANOVA with Newman-Keulspost-hocanalyses was used for comparisons. Data are mean±s.e.m. for 20 cells from five monolayers for each group. Figure 5: Dextran permeation through endothelial adherens junctions. ( a , b ) Confocal images of WT endothelial monolayers show dextran permeation. ( a ) The left image shows an x – y projection of an endothelial cell of a monolayer expressing full-length GFP-cad (blue pseudocolor). The cytosol is stained with calcein red. The right image shows the x – z projection of an HAJ identified at the cross-hairs on the left image. Ap, apical; BI, basolateral. ( b ) After layering dextran of 4 (D4), 20 (D20) or 70 (D70) kDa (green) on the apical surface, fluorescence accumulation in the x – z plane was imaged over time. D4 and D20, but not D70 penetrated the HAJ. Red pseudocolor denotes the cytosol. Rectangles show sites of analyses for dextran fluorescence in the junctional cleft. ( c , d ) Plots from single AJs and the group data show time course of dextran accumulation. Scale bars are 10 μm ( x – y images) and 2 μm ( x – z images). *P<0.005 compared with HAJ of D4, †P<0.005 compared with LAJ of D20 and $P<0.005 compared with HAJ of D20. ( e ) Group data for LAJs and HAJs show D70 penetrance at 30 min for monolayers transfected with full-length (FL) or mutant (W2A) E-cadherin or with the α-actinin-1 mutant (Y12F). * P <0.002 compared with left bar. $ P <0.002 compared with HAJ in WT group. ANOVA with Newman-Keuls post-hoc analyses was used for comparisons. Data are mean±s.e.m. for 20 cells from five monolayers for each group. Full size image To determine whether these sieving properties were differentially regulated by ectodomain versus actin interactions of cadherin, we assayed D70 penetrance in monolayers expressing the Y12F or W2A mutants ( Fig. 5e ). Shaking-bath assays on isolated, mutant-expressing endothelial cells indicated that both mutants inhibited cell aggregation ( Fig. 6a–c ). This lack of aggregation in isolated cells did not abrogate monolayer cohesiveness, as endothelial cells expressing these mutants were able to form continuous monolayers in which HAJ distribution profiles were similar to WT ( Figs 2b and 3c ). However in the presence of the Y12F or W2A mutation, D70 penetrance at HAJs increased markedly such that it was not different from the D70 penetrance in WT LAJs ( Fig. 5e ). Interestingly, the mutants did not increase D70 penetrance above WT levels at LAJs, indicating that strand–swap and actin-bundling effects in sieving were restricted to HAJs. As we discuss above, the W2A mutation did not change actin distribution, we interpret that the W2A mutation caused actin-independent loss of sieving at HAJs. 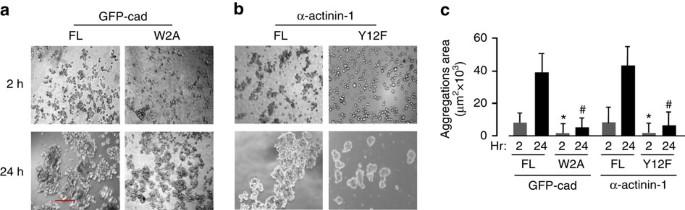Figure 6: Endothelial aggregations by the shaking bath assay. (a,b) Images show isolated endothelial cells expressing full-length (FL) or mutant (W2A) E-cadherin and α-actinin-1 mutant (Y12F) were exposed to 2 or 24 h in a shaking bath. (c) Group data of aggregation assay for corresponding monolayers . Data are mean±s.e.m. from four monolayers for each group. *P<0.005 compared with 2 h data point in WT group; #P=0.001 compared with 24 h data point in WT group. ANOVA with Newman Keulspost-hocanalyses was used for comparisons. Scale bar, 200 μm. Figure 6: Endothelial aggregations by the shaking bath assay. ( a , b ) Images show isolated endothelial cells expressing full-length (FL) or mutant (W2A) E-cadherin and α-actinin-1 mutant (Y12F) were exposed to 2 or 24 h in a shaking bath. ( c ) Group data of aggregation assay for corresponding monolayers . Data are mean±s.e.m. from four monolayers for each group. * P <0.005 compared with 2 h data point in WT group; # P =0.001 compared with 24 h data point in WT group. ANOVA with Newman Keuls post-hoc analyses was used for comparisons. Scale bar, 200 μm. Full size image Cadherin mobility correlates with macromolecular sieving As our findings implied that endothelial mutations that increased cadherin mobility at HAJs also increased 70 kDa dextran penetrance, we determined the relationship between AJ mobility and dextran permeability in the presence of physiological barrier regulators. Hyperosmolar sucrose increases [12] , whereas H 2 O 2 decreases endothelial barrier properties [41] , [42] , [43] . Consistent with these known overall barrier responses, these agents induced different segment-specific changes in D70 penetrance in that hyperosmolar sucrose decreased the penetrance at LAJs, whereas H 2 O 2 increased the penetrance at HAJs ( Fig. 7a ). Concomitantly, cadherin mobility responses were also segment specific in that hyperosmolar sucrose decreased the mobile fraction at LAJs ( Fig. 7b ), whereas H 2 O 2 increased the mobile fraction at HAJs ( Fig. 7b ). Further, cadherin density in the endothelial junction increased in the presence of hyperosmolar sucrose ( Fig. 7c ), but it decreased after H 2 O 2 exposure ( Fig. 7d ). The cumulative plot of cadherin mobile fraction against dextran 70 penetrance at HAJs revealed a linear relationship ( Fig. 7e ), suggesting that cadherin mobility is a determinant of macromolecular sieving. 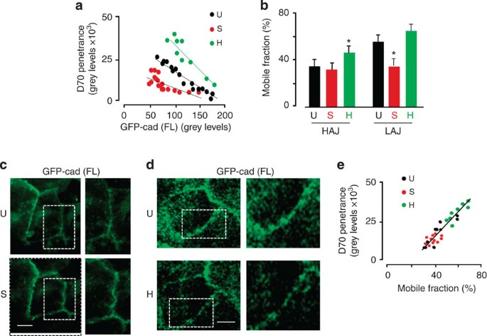Figure 7: Effects of barrier modifying agents on endothelial HAJs. Endothelial monolayers were exposed to hyperosmolar sucrose (S) or H2O2(H) for 30 min. Responses in these and untreated (U) monolayers are shown as the D70 penetrance–AJ density relation (a), and the cadherin mobile fraction (b). The lines were drawn by linear regression (P<0.05 for each line). *P<0.001 compared with the untreated group. Significance was calculated by two-tailed pairedt-test. Data are mean±s.e.m. for 50 cells from four monolayers for each group. (c,d) Confocal images show monolayers expressing full-length GFP-cad (GFP-cad FL). The right images in each set are magnifications of the demarcated regions (rectangles). The endothelial responses shown in the lower images were obtained 30 min after sucrose or H2O2exposure. (e) The data fromaandbare plotted as shown. The relationship is significant atP<0.05 as determined by linear regression (30 cells from four monolayers in each condition). Figure 7: Effects of barrier modifying agents on endothelial HAJs. Endothelial monolayers were exposed to hyperosmolar sucrose (S) or H 2 O 2 (H) for 30 min. Responses in these and untreated (U) monolayers are shown as the D70 penetrance–AJ density relation ( a ), and the cadherin mobile fraction ( b ). The lines were drawn by linear regression ( P <0.05 for each line). * P <0.001 compared with the untreated group. Significance was calculated by two-tailed paired t -test. Data are mean±s.e.m. for 50 cells from four monolayers for each group. ( c , d ) Confocal images show monolayers expressing full-length GFP-cad (GFP-cad FL). The right images in each set are magnifications of the demarcated regions (rectangles). The endothelial responses shown in the lower images were obtained 30 min after sucrose or H 2 O 2 exposure. ( e ) The data from a and b are plotted as shown. The relationship is significant at P <0.05 as determined by linear regression (30 cells from four monolayers in each condition). Full size image Our findings indicate that the transport of large macromolecules across the endothelial barrier is regulated by HAJs and LAJs that are, respectively, restrictive and permissive to macromolecular transport. This arrangement reduces the total surface area of junctional penetrance for large molecules of the size of 70-kDa dextran, which are restricted to the LAJs, whereas smaller molecules have transport access through both LAJs and HAJs. According to the current understanding of endothelial sieving, differences in junctional geometry or the presence of an apical fibre matrix determine differential restriction to protein transport [2] , [3] . Our findings suggest on the other hand, that endothelial sieving results mainly from the spatial distribution of HAJs. The W2A mutation caused no impairments in the F-actin density distribution, indicating that loss of the strand–swap interactions had no significant impact on the cortical actin cytoskeleton. In W2A-expressing monolayers, although the AJ clustering pattern was similar to that of untransfected cells, cadherin mobility increased two times above control. Hence, to the extent that F-actin density was preserved at the HAJs, our findings indicate that loss of the strand–swap interactions was sufficient to increase cadherin mobility. We suggest therefore that at endothelial HAJs, cadherin tethering is critically determined by adhesive-binding interactions between cadherin EC1 domains of adjoining cells. Although multiple reports attest to the F-actin role in the maintenance of the endothelial barrier [20] , [30] , [44] , the manner in which F-actin regulates AJs is not clear. As the actin-bundling protein, α-actinin-1, co-distributed with F-actin at HAJs, we expressed the Y12F mutation to decrease F-actin binding to α-actinin-1. In Y12F-expressing monolayers, F-actin loss was specific to HAJs, indicating that the F-actin accumulation at HAJs was α-actinin-1 dependent. In epithelia, at least two pools of cortical F-actin are described, namely the latrunculin-sensitive and -insensitive pools [31] . Other evidence for multiple actin pools comes from micromechanical analyses by atomic force microscopy. These studies indicate the presence of F-actin containing coarse and fine meshes [45] that account for local differences in elastic modulus [46] , [47] . The increased viscosity attributable to actin bundling might provide mechanical stability to HAJs. The Y12F mutation decreased, but did not completely eliminate F-actin from HAJs. We suggest that the loss of sieving due to the Y12F mutation resulted from loss of the cadherin anchorage through α-actinin-1. Our novel dextran penetrance studies provided an understanding of the site-specific dextran permeability at the LAJs and the HAJs. The extent of tracer penetrance in the endothelial junction is probably best characterized by determining tracer concentration at the site at which the tracer exits the junction on the basolateral aspect of the cell. However, this determination was not possible, as tracer exiting the junction at the HAJs mixed with tracer exiting the LAJs, making site-specific penetrance determinations difficult. Hence, we obtained the penetrance determinations at a site proximal to the junction exit. To confirm that the junctions were patent, we determined penetrance of 4 kDa dextran (D4). As D4 has a molecular diameter of about 1 nm, the endothelial barrier is not expected to impede its transit. Consistent with this expectation, D4 penetrated both LAJs and HAJs rapidly and completely. We conclude that although HAJs contain channels that accommodate transit of small molecules of molecular size equal to or less than that of D4, the channels impede molecules of size equivalent to or greater than D70. The importance of cadherin adhesive binding between cells on endothelial sieving was revealed by the dextran penetrance assay. Although the W2A mutant blocks aggregation of isolated cells, a finding we confirmed by the shaking-bath assay, expression of the W2A mutant did not compromise overall cell adhesion in the monolayer, as indicated by the maintenance of the transendothelial electrical resistance. Despite this evidence for overall cell cohesion, the penetrance assay revealed marked differences in permeability to 70 kDa dextran between WT and W2A monolayers in that WT HAJs almost completely excluded the dextran, whereas W2A HAJs were highly permeable. The optical data indicate that endogenous cadherin was equally well expressed at the junctions in non-transfected versus W2A-overexpressing cells, ruling out cadherin density as a factor in the penetrance response. These findings indicate that the strand–swap interaction in cadherin EC1 domain, which the W2A mutation abrogated, was the critical factor that determined the D70 restriction at HAJs. It is likely that the high cadherin density at HAJs increases clustering of strand–swap interactions, thereby narrowing local fluid channels. Our findings suggest that the extent of cadherin mobility at HAJs associates with the extent of macromolecular penetrance. A comparison of the W2A and the Y12F monolayers indicated that the increases in cadherin mobility and in D70 penetrance occurred to a similar extent in both. These similarities suggest that from the standpoint of macromolecular sieving, the hyperpermeability effect of depleting F-actin at HAJs was more or less equivalent to that of blocking strand–swap interactions. The barrier significance of cadherin mobility was revealed through dextran penetrance at HAJs in the presence of barrier-modifying agents. Peroxide reduces F-actin and decreases the endothelial barrier [48] , [49] . Hyperosmolar sucrose has the opposite effect [12] . The mobility and penetrance effects were consistent with these expectations. Hyperosmolar sucrose, which mainly tightened the barrier at the LAJs, decreased both cadherin mobility and D70 penetration across the entire junction. H 2 O 2 , which increased HAJ permeability, increased the overall junctional permeability. Consistent with the notion that cadherin packing determines these responses, hyperosmolar sucrose increased, whereas H 2 O 2 decreased junctional cadherin. A pooled plot of measurements for all groups obtained at different junctional microdomains revealed a strong linear correlation between dextran penetrance and cadherin mobility, indicating that increased cadherin mobility, presumably due to loss of EC1 trans interactions, associates with decreased sieving at HAJs. In consideration of the fact that our findings in non-confluent monolayers indicate that LAJs can remodel to form HAJs and vice versa, we suggest that with hyperosmolar sucrose LAJs transformed to HAJs, whereas the opposite occurred with H 2 O 2 . The biological significance of our findings relates to the manner in which endothelial cells regulate transvascular mass transport. A long-standing debate addresses the transport route that could entail transcytosis, a process by which endothelial plasmalemmal vesicles, or caveolae, shuttle proteins from blood to interstitium [50] , or passive paracellular transport [51] . Although the relative contributions of the two pathways to total transport remain unclear, the paracellular pathway is thought to regulate the transport by reorganizing the actin cytoskeleton, as for example, to subserve the pro-permeability effects of H 2 O 2 [42] . However, the effects of such cytoskeletal reorganization on AJ cadherin linkages remains unclear. We propose that the paracellular component might be determined by the distribution of HAJs and LAJs that, respectively, provide the protein-restricting and -permissive regions of the junction. Although these findings need to be confirmed in vivo , we suggest that by modulating the relative distributions of HAJs and LAJs, an effect that was induced here by hyperosmolar sucrose and H 2 O 2 , the endothelial cell regulates the overall permeability of the paracellular pathway. In summary, we show here that the cadherin interactions at the EC1 domain as well as with cortical F-actin are important for the sieving properties of the endothelial barrier. A key result was that despite the fact that the two mutants used here addressed completely different junction assembly mechanisms, namely those involving EC1 interactions and F-actin density, the net effects on cadherin stability and macromolecular penetrance were similar. The higher macromolecular penetrance and higher cadherin mobility at the LAJs and the Y12F-expressing HAJs suggests that at WT HAJs, F-actin localizes AJ-forming proteins at high density to construct a barrier with low macromolecular penetrance. The equal increases of D70 penetrance and cadherin mobility at HAJs with both mutants suggests that a critical density of F-actin as well as EC1 interactions together maintain the stability of the HAJs, hence the selectivity properties of the barrier. Reagents Plasmids: the plasmid vector for WT mouse E-cadherin (NM_009864) was a gift of Dr Kusumi (Nagoya University, Japan) [52] . The plasmid vector for WT α-actinin (X15804) and the mutant Y12F were gifts of Dr Haimovich (RWMS UMDNJ, New Jersey) [53] . The plasmid for the E-cadherin mutant W2A was generated by site-directed mutagenesis of WT E-cadherin to replace the second tryptophan (W) to alanine (A) in ectodomain-1 (QuikChange, Stratagene). To obtain fluorescent, hygromycin-expressing constructs, we generated the backbone vector mOrange2-hyg-N. Then we released α-actinin-1 or Y12F from the original vector and inserted these segments into the backbone vector at the Hind II/ Age I site to yield α-actinin-mOrange2-hyg-N and Y12F-mOrange2-hyg-N plasmid vectors. DNA sequencing was performed to confirm the correct introduction of the mutations (Genewiz). Chemicals: Chemicals were obtained from Sigma, unless otherwise stated. Anti-α-catenin rabbit polyclonal Ab, anti-β-catenin mAb, anti-phosphotyrosine mAb PY99 (mouse, monoclonal), anti-F-actin antibody (goat), protein A/G-agarose beads and horseradish peroxidase-linked anti-mouse or anti-rabbit Ig Ab were purchased from Santa Cruz. Anti-E-cadherin mAb (BD Biosciences) and Alexa 488-conjugated phalloidin (Invitrogen) was used for staining actin filaments. Cell culture media, M199 medium, gentamycin (G418, 100 μg ml −1 ) and Opti-MEM, lipofectin and antibiotics (50 U ml −1 penicillin G and 50 μg ml −1 streptomycin) were obtained from Invitrogen. All reagents for immunofluorescence studies were obtained from Molecular Probes (Eugene). Cell culture, transfection and protein analysis Rat lung microvascular endothelial cell (RLMEC) were cultured as described under standard conditions and transfected using Lipofectin (Invitrogen) [12] . We selected colonies by growing cells in G418-containing medium that allows growth of only transfected cells, then sorting for GFP- or mOrange2-positive cells (BD FACS Aria Cell Sorter). Cells were plated at a density of 10 5 per cm 2 . The endothelial cell phenotype was confirmed by cell uptake of fluorescein-tagged acetylated-low-density lipoprotein (DiI-Ac-LDL) as detected by optical imaging. Immunoprecipitation, immunoblotting and surface E-cadherin expression were performed as described previously [12] , [42] . Detection of surface protein expression Endothelial monolayers were grown on 100 mm cell culture plates. Plates were placed on ice and exposed to biotin for 1 h (1.5 mg ml −1 , sulfo-NHSSS-biotin; Pierce, Rockford, IL), followed by a wash with blocking reagent (50 mM NH 4 Cl in PBS containing 1 mM MgCl 2 and 0.1 mM CaCl 2 ) to remove free biotin. After several washes with PBS, cells were lysed in buffer (300 μl, 25 mM Tris–HCl pH 7.4 with 150 mM NaCl, 0.1% SDS, 1% Triton X-100 and 1% deoxycholate) containing protease inhibitors (Roche Molecular Biochemicals, Mannheim, Germany). The cell lysate was clarified by centrifugation at 10,000 g for 10 min. Protein concentrations were determined using a protein analysis kit (BCA, Pierce). Equal amounts of protein were incubated with streptavidin beads (Sigma) to bind biotinylated proteins (4 μg, 2 h; BD Biosciences) and the mixture was incubated overnight at 4 °C. Precipitates were recovered by centrifugation. Non-specific proteins were removed by washing the agarose beads with cell lysate buffer and PBS. Bound proteins were recovered from the beads in protein-elution buffer (Pierce), then resolved by SDS-polyacrylamide gel electrophoresis. After transfer to nitrocellulose membranes, the proteins were analysed by immunoblotting (antibody concentration, 0.2 μg ml −1 ). Band densities were analysed by densitometry (Image station 4000MM, Kodak Scientific Imaging Systems, Rochester, NY). Cell fractionation for G-actin and F-actin A two-step solubilization of F-actin was carried out [12] . In this approach, we used a mild solubilizing buffer to extract G-actin in the supernatant of the clarified sample. The stronger solubilizing buffer was then applied to the pellet to extract F-actin. Cells were rinsed 2× PBS and solubilized in mild lysis buffer (50 mM NaCl, 10 mM Pipes, pH 6.8, 3 mM MgCl 2 , 0.05% Triton X-100, 300 mM sucrose, 1 μg ml −1 leupeptin, 1 μg ml −1 aprotinin, 1 mM phenylmethylsulfonyl fluoride) for 20 min at 4 °C on a rocking platform. The cells were scraped from the plate and centrifuged (10 min). The supernatant was collected (Triton soluble). The cell pellet was suspended in 100 μl of stronger solubilizing buffer (15 mM Tris, pH 7.5, 5 mM EDTA, 2.5 mM EGTA, 1% SDS 1 μg ml −1 leupeptin, 1 μg ml −1 aprotinin, 1 mM phenylmethylsulfonyl fluoride) and boiled for 10 min to dissolve the pellet and then diluted to 300 μl with RIPA buffer. Equal amounts of extracted proteins were loaded for SDS–PAGE gel electrophoresis. Band densities were quantified by densitometry as above. Immunofluorescence microscopy Fixed samples were processed conventionally for immunofluorescence microscopy as described [12] , [42] , [54] . Endothelial monolayers plated on glass coverslips were fixed using 4% paraformaldehyde and permeablized by 0.1% Triton X-100 for 5 min. Fixed cells were incubated with blocking solution (1 h, 25 °C) and then with primary antibodies (10 μg ml −1 ) followed by appropriate secondary antibodies (10 μg ml −1 ) coupled to either Alexa 488 or Alexa 568 (Invitrogen). PBS washes (3×5 min each) were performed between all steps and images were captured by confocal microscopy (LSM 510 Meta, Zeiss). Permeability measurement Live monolayers were stained with the cytosolic dye, calcein red (5 μM ml −1 ; for 10 min). FITC-labelled dextrans of different molecular sizes, namely 4 (D4), 20 (D20) and 70 kDa (D70) were added on the apical aspects of the monolayers. The monolayers were then imaged by confocal microscopy at 37 °C at different time points as stated. Apical to basolateral transport of dextran-FITC was assessed in the x – z plane of inter-endothelial clefts. Dextran concentration was calculated from the fluorescence data using calibration curves established with dextran-FITC stock solution. The data were analysed by imaging software (Metamorph 6.3, Universal Imaging, Downington, PA). Fluorescence recovery after photobleaching (FRAP) FRAP measurements were performed by confocal microscopy (LSM 510 Meta, Zeiss). Several regions of the membrane were photobleached simultaneously by argon laser (488 nm) throughout the cell depth, as confirmed by Z-stack images. We monitored fluorescence recovery by scanning the bleached area with an attenuated laser beam (5% power). To rule out non-specific bleaching, we corrected the fluorescence recovery against non-bleached regions of the image. Kymographs show the FRAP time course. The mobile fraction was determined as described [55] . The mobility (% of FRAP) was calculated after subtracting non-specific fluorescence from the total fluorescence intensity. The non-specific fluorescence was determined as the fluorescence of a reference site not exposed to photobleaching. The mobile fraction was determined as ( F ∞− F o)/( F i− F o), where F ∞ is the fluorescence in the bleached region after fluorescence recovery at infinite time, F i is the fluorescence before bleaching and F o is the fluorescence immediately after bleaching [55] . The recovery curves were fit to the equation y = yo + a (1– e − kt ), where k is the rate constant and t ½ is the half-time to full fluorescence recovery. k was calculated by nonlinear regression (exponential rise to maximum; three parameters) without any constraints using graphing software (Sigma Plot, Systat Software Inc.). Confocal microscopy and image analysis Confocal images were obtained by laser scanning microscopy as we published previously [54] (LSM 510, Zeiss, Thornwood, NY). GFP and mOrange were excited using the 488-nm laser line of an argon laser and the 543-nm laser line of a helium-neon laser, respectively. Single plane and Z-stack images were taken using ×40 water-immersion objectives. Image acquisition and analyses were carried out using software (LSM image browser, Zeiss; Metamorph, Universal Imaging, Media, PA). Aggregation assay We used two types of aggregation assays to assess specificity of cadherin adhesion, namely the short-term and the long-term assays [26] . The short-term assay utilizes cell-culture medium in Hanks balanced salt solution containing 1% bovine serum albumin in a volume of 0.5 ml. This assay has a time-course of 2 h with cell mixing generated through orbital shaking at 70 r.p.m. The long-term assay is similar, except the shaking is carried for 24 h. Data analysis Fluorescence data reflect analyses on 60–80 cells per experiment from 4–6 experiments. Group data are presented as mean values±s.e.m. All group data were obtained from experiments repeated in separate monolayer unless otherwise stated. Statistical data analysis was performed using Sigma Plot (Systat Software Inc.). Paired comparisons were by the paired t -test and multiple comparisons by one-way ANOVA followed by Newman-Keuls post-hoc analysis. We accepted significance at P <0.05. How to cite this article: Quadri, S.K. et al . Cadherin selectivity filter regulates endothelial sieving properties. Nat. Commun. 3:1099 doi: 10.1038/ncomms2107 (2012).